Creation of a gated antibody as a conditionally functional synthetic protein The ability to conditionally direct antibodies is a potentially powerful application for Synthetic Biology in Medicine. Here we show that control of antibody binding through site-specific, chemical phosphorylation of a recognition domain creates a ‘gated’ antibody (Ab). This displays a crude Boolean logic where binding is induced in an enzyme-AND-antigen dependent manner. This ‘AND-Ab’ is therefore active only in the presence of two biomarker inputs: the simultaneous expression of a (cell surface) antigen and secreted enzyme to generate function in vitro , on cells and in mammalian tissue. Such gated Abs, either alone or in combination, could allow the application of logic strategies to enhance precision in biological interrogation, modulation and in therapy. One of Synthetic Biology’s goals is to create biological units (biobricks [1] ) with a reductionist and standardized behaviour that will enable greater reliability in application and exploitation [1] . However, the exploitation of such strategies in systems of translational relevance to medicine has been limited. To date, artificial, gated biological systems have been developed that exploit nucleic acids. Many operate at a genetic level, where the precise and tuneable control of gene expression (inputs) leads to selected protein synthesis outputs [2] , [3] , [4] , [5] , [6] , [7] . In this way, ‘AND’ gating, where a function is reliant on the presence of multiple inputs, has emerged as a potential strategy for the targeted control of cellular protein synthesis [8] and growth inhibition of tumour cells [9] . However, as a result of the time ‘lag’ generated by intervening transcriptional and translational processes, expression-based gates display slow response times that may not be suitable for highly dynamic biological environments, such as at cell surfaces or in tissues. Moreover, DNA-based constructs have been developed for conditional delivery of payloads based on an antigenic ‘input’ [10] . Yet, the susceptibility of exposed nucleic-acid based ‘robots’ to nucleases in vivo would prevent widespread application. For these situations and others, the potentially rapid responses of stable protein ‘gates’ would be preferable. A vision [11] for diverse protein-based computation, and in particular its application to useful medicinal strategies, is therefore far from complete. Given the pivotal role of proteins as the workhorses of Biology, such conditionally functional or ‘gated’ proteins could be powerful tools with diverse roles in Medicine. One family of protein motifs with particular power are the phosphorylated amino acids due to their binary, toggle-like states (phosphorylation or not) and the dramatic functional effect that this single residue switching can have even upon large proteins [12] . A second protein motif type with specific, input-like behaviour are the complementarity determining regions (CDRs) of antibodies that mediate binding as an output upon display of an antigen input. To the best of our knowledge, nature has never combined these two powerful elements of protein control; we reasoned that such multi-input processing by a protein could create a protein ‘state engine’ as a gated system with a wide range of potential applications ( Fig. 1 ). No current phosphorylating enzyme has yet been demonstrated to be capable of modifying Ab CDRs. 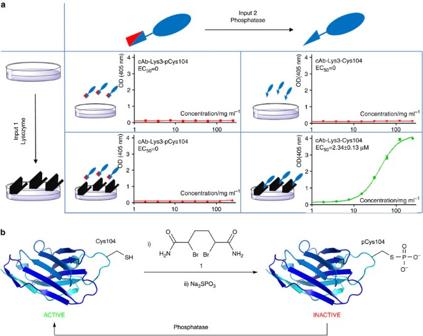Figure 1: Design and construction of a ‘gated’ antibody. (a) The gated two-input activation of an AND antibody based upon cAbLys3. Input 1 is presentation of the corresponding selective antigen (black shape, here lysozyme) that engages as a ligand for the Complementarity Determining Region (CDR) in its unblocked state. Input 2 is the presence of the enzyme that unblocks that CDR by removing a blocking group (red shape, here removed by phosphatase). Enzyme-linked immunosorbent assay data for binding shows functional ‘output’ only upon the presence of both inputs (green). All other input states fail to generate activity (red). (b) The gated AND antibody that responds to this input can be constructed in a highly stable, single-chain form through site-selective, chemical phosphorylation within the CDR to block its binding function. Active cAbLys3 containing an engineered Cys residue at residue 104 (A104C) was reacted first with the HDADB reagent (1) to create unnatural amino acid Dha (step i) and then with sodium thiophosphate (step ii) to introduce phosphoryl as a blocking group thereby rendering the Ab inactive. The phosphoryl block group is removed by the action of phosphatase-catalyzed dephosphorylation to unblock the CDR and regenerate active antibody binding as an output. Figure 1: Design and construction of a ‘gated’ antibody. ( a ) The gated two-input activation of an AND antibody based upon cAbLys3. Input 1 is presentation of the corresponding selective antigen (black shape, here lysozyme) that engages as a ligand for the Complementarity Determining Region (CDR) in its unblocked state. Input 2 is the presence of the enzyme that unblocks that CDR by removing a blocking group (red shape, here removed by phosphatase). Enzyme-linked immunosorbent assay data for binding shows functional ‘output’ only upon the presence of both inputs (green). All other input states fail to generate activity (red). ( b ) The gated AND antibody that responds to this input can be constructed in a highly stable, single-chain form through site-selective, chemical phosphorylation within the CDR to block its binding function. Active cAbLys3 containing an engineered Cys residue at residue 104 (A104C) was reacted first with the HDADB reagent ( 1 ) to create unnatural amino acid Dha (step i) and then with sodium thiophosphate (step ii) to introduce phosphoryl as a blocking group thereby rendering the Ab inactive. The phosphoryl block group is removed by the action of phosphatase-catalyzed dephosphorylation to unblock the CDR and regenerate active antibody binding as an output. Full size image Here we circumvent this limitation in Biology through the use of a site-selective, chemical phosphorylation strategy. Site-selective chemical modification of proteins allows the introduction of both natural and non-natural functionalities with potentially near-unlimited control of site and alteration. The ‘tag-and-modify’ approach involves the introduction of an orthogonally reactive functional group —the tag— that can be used as a selective chemical handle for further modification and introduction of the desired group [13] . In particular, the incorporation of dehydroalanine (Dha) as a tag allows diverse modification [14] . Here, we use this mode of synthetic protein construction to assemble such a gated, ‘multi-input’ protein ( Fig. 1 ). Design and Construction of a Gated Antibody Position 104 in the CDR3 loop of the single-domain antibody cAb-Lys3 (refs 15 , 16 ) was chosen as a pivotal residue in the CDR3 loop that is key for hydrophobic interaction with the model cognate antigen lysozyme [16] . We thus chose to sublocate a phosphorylation site within the CDR and, in this way, colocalize the region for two protein inputs (antigen and phospho-state) that would putatively control output (binding). The creation of a polar group at a site used normally to mediate hydrophobic interactions was intended to logically exploit a suggested evolved ‘switching’ mechanism of phosphorylation state [12] . A Dha ‘tag’ was site-selectively installed at position 104 by treating cAbLys3-Cys104 with selective reagent 1 ( Fig. 1b(i) , ref. 14 ) followed by reaction with sodium thiophosphate to create the phospho-amino acid phosphocysteine (pCys) ( Fig. 1b(ii) ) in cAbLys3-pCys104. The reactions proceeded cleanly and completely ( Supplementary Results , Supplementary Figs 1–3 ). Protein characterization confirmed generation of the intended folded protein cAbLys3-pCys104: peptide mapping using proteolytic digestion and liquid chromatography-mass spectrometry (LC-MS)/MS confirmed that the modification occurred at position 104 only ( Supplementary Figs 4–6 ), despite the presence of other native cysteines in disulphide bonds thereby highlighting selectivity. Circular dichroism revealed that cAbLys3-pCys104 retained its largely β-sheet structure ( Supplementary Fig. 7 ). Enzyme-linked immunosorbent assay showed that antigen (lysozyme) binding ability was dramatically inhibited ( Fig. 1a , bottom left). In this way the resulting antibody was rendered incapable of binding (output) upon presentation of only a single input (antigen). Testing a Second Input to Demonstrate AND-Ab Activity We next investigated the effect of controlling the second input, phosphorylation state. We treated antibody cAbLys3-pCys104 with a range of phosphatases as natural, enzymatic modulators of phospho-state. O -phosphate group removal (particularly at threonine, serine and tyrosine residues) is not only an excellent modulator of protein state but phosphatases are imperative to a myriad of cellular processes in the body [17] . This form of input to our synthetic multi-state protein might therefore also serve as a ‘read-out’ or biomarker of many current cellular processes. cAbLys3-pCys104 contains an S -linked analogue phospho-aminoacid (phosphocysteine, pCys) of the more usual, natural substrate phospho-serine (pSer). Although many protein phosphatases are suggested to be promiscuous [17] , [18] , reports regarding S -linked phosphate group removal are uncommon in eukaryotes and cysteine phosphorylation is considered rare, although its occurrence and important regulatory roles in bacteria are being explored [19] . We discovered that not only could the phosphate group of cAbLys3-pCys104 be cleaved by a range of different phosphatases in ambient conditions to regenerate cysteine at position 104 of cAbLys3-Cys104 ( Supplementary Figs 8–12 ) but also that, when so treated with phosphatase, binding ( Fig. 1a , bottom right) with constants in a similar range to that of the original cysteine mutant were obtained ( Supplementary Fig. 13 ). Thus, only in the presence of two inputs (antigen lysozyme+enzyme phosphatase, Fig. 1a ) was function obtained; the synthetic antibody cAbLys3-pCys104 may therefore be considered to be an ‘AND antibody’ (AND-Ab). This activated synthetic AND-Ab was fully characterized by MS, peptide mapping (proteolytic digestion and MS/MS) and spectroscopic analysis using Ellman’s reagent, which confirmed the presence of free Cys104 ( Supplementary Fig. 14 ). The relative efficiencies of phosphatase-mediated pCys→Cys switching as an input in cAbLys3-pCys104 at physiological pH and temperature were directly investigated, with an interest to application in organismal or therapeutic settings. This revealed that under identical conditions cAbLys3-pCys104, interestingly, showed different relative sensitivities to different representative phosphatase enzyme subtypes. In particular, efficient and rapid cleavage could be obtained even with low levels of several forms of alkaline phosphatase, including bovine intestinal mucosa phosphatase and human placenta alkaline phosphatase (huPLAP, Supplementary Figs 15–20 ). Notably, the latter is found in variously truncated forms in different human tissue types and is known to report on cell type and state (a putative biomarker) [20] . Cellular Application of the AND-Ab Next, we tested the interaction of the AND-gated Ab in a cellular context. The AND-Ab is designed to be activated by two inputs that, in principle, could be found at a cell surface or extracellularly, thereby allowing potential exploitation of this strategy in valuably relevant complex biological contexts. Two human cellular systems (using human embryonic kidney (HEK293T) cells) were constructed that would test this principle ( Fig. 2a ) capable of controllable generation of the two inputs needed by the AND-Ab: the cell-surface display of antigen (lysozyme), and the secretion of enzyme (phosphatase). To generate the antigen input under the control of these cells, the gene encoding for expression and cell-surface localization of lysozyme ( lys ) under the control of a CMV promoter was obtained using vector pIMMs2011LysD52S (see Supplementary Methods ). Transfection of HEK cells with the lys gene (using a poly(β-amino ester) transfection agent, Xfect, (Clontech)) generated cell-surface display of lysozyme in HEK293- lys+ cells; this was confirmed by flow cytometric analysis of the binding of WT-cAbLys3 (ref. 16 ), detected using a fluorescently-labelled (Alexa Fluor 488) secondary Ab ( Supplementary Fig. 21 ). To generate the enzyme (phosphatase) input under the control of these cells, secreted embryonic alkaline phosphatase (SEAP) [20] , [21] was expressed in HEK293- seap+ cells (using Xfect-mediated transfection by a pBluescript vector containing CMV- seap , Addgene, plasmid 24595). SEAP was chosen as a form of huPLAP that lacks the membrane-anchoring domain, and is therefore secreted by cells, potentially allowing extracellular control. HuPLAP had been previously identified as an excellent input for the AND-Ab (see above) and showed excellent thiophosphate cleavage activity on cAbLys3-pCys104 and hence input ability for the AND-Ab ( Supplementary Fig. 8 ). 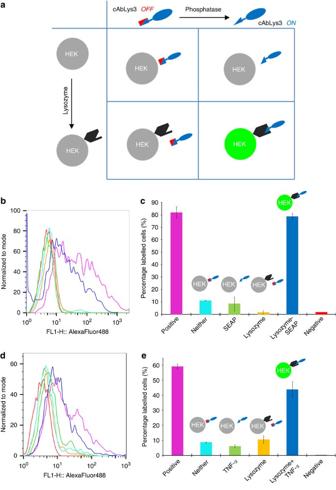Figure 2: Cell surface gated activation of the AND antibody. (a) Anin vitroAND-gated antibody can be directed to bind to a cell surface only in the presence of two inputs. (b,c) Flow cytometry traces and corresponding percentage of labelled cells for inhibited antibody added to HEK cells expressing different input combinations. A higher percentage of labelled cells is observed where inhibited antibody is added to cells expressing both cell surface lysozyme and secreted phosphatase as inputs (HEK-lys+-seap+ cells, dark blue). Positive control (shown in pink) is cAbLys3 wild type added to cells expressing cell surface lysozyme. The differences to other conditions can be seen clearly. (d,e) The AND-Ab also responds to indirect triggering of inputs. Relaying of an indirect TNF-α cytokine signal using HEK cells (HEK-Blue Null1 (NFκB-seap+) HEK293T cells stably expressing NF-κb-inducible SEAP reporter construct under IFN-β minimal promoter) generates the SEAP input only under the indirect control of stimulation by the IFN-β minimal promoter. In this more complex cellular system, the AND-Ab shows a similar trend in its significant response to the dual inputs. Error bars were calculated using the s.d. of measurements taken in triplicate. Figure 2: Cell surface gated activation of the AND antibody. ( a ) An in vitro AND-gated antibody can be directed to bind to a cell surface only in the presence of two inputs. ( b , c ) Flow cytometry traces and corresponding percentage of labelled cells for inhibited antibody added to HEK cells expressing different input combinations. A higher percentage of labelled cells is observed where inhibited antibody is added to cells expressing both cell surface lysozyme and secreted phosphatase as inputs (HEK- lys +- seap + cells, dark blue). Positive control (shown in pink) is cAbLys3 wild type added to cells expressing cell surface lysozyme. The differences to other conditions can be seen clearly. ( d , e ) The AND-Ab also responds to indirect triggering of inputs. Relaying of an indirect TNF-α cytokine signal using HEK cells (HEK-Blue Null1 ( NFκB-seap +) HEK293T cells stably expressing NF-κb-inducible SEAP reporter construct under IFN-β minimal promoter) generates the SEAP input only under the indirect control of stimulation by the IFN-β minimal promoter. In this more complex cellular system, the AND-Ab shows a similar trend in its significant response to the dual inputs. Error bars were calculated using the s.d. of measurements taken in triplicate. Full size image The AND-Ab was tested against human cells generating a combination of these two inputs (expression of cell-surface lysozyme and/or SEAP; Fig. 2a ). The proper generation of these inputs by the cells was confirmed using WT-cAbLys3 (to show generation of antigen input, Fig. 2b,c , pink trace) and chromophoric phosphatase substrate (to show generation of antigen input, Supplementary Results , Supplementary Figs 22,23 ). When added to the supernatant, the AND-Ab responded only to the two inputs (see Fig. 2a ) from these human cells, as measured by fluorescence-activated cell sorting cytometric analysis ( Fig. 2b,c ). Gratifyingly, 79% of cells generating both lysozyme and SEAP as biomarkers were detected, near identical to the level obtained in positive controls using WT-cAbLys3 under identical conditions (82% labelled cells, see Fig. 2b,c , dark blue). The absence of one or both inputs led to a dramatic decrease in detection ( Fig. 2b,c ), consistent with the gated AND-Ab design. In these HEK- lys +- seap + cells the cell-generated inputs were under direct control. In complex biological systems, relevant biomarkers and messengers may be generated indirectly. To test the relaying of such indirect signals, HEK293T cells (HEK-Blue Null1 ( NFκB-seap +) stably expressing an NF-κb-inducible SEAP reporter construct under IFN-β minimal promoter) that generate the SEAP input only under the indirect control of stimulation by the IFN-β minimal promoter fused to five NF-κB and AP-1 binding sites were used. In this more complex cellular system, SEAP expression (and this input) can therefore be induced by the addition of the cytokine TNF-α, a mammalian messenger molecule with widespread signalling function in disease states [22] . This control mechanism was confirmed by test of resulting phosphatase activity, using again chromophoric phosphatase substrate ( Supplementary Fig. 24 ). The AND-Ab was then tested against these human cells under indirect stimulation of TNF-α (100 ng ml −1 ); only in the presence of both inputs, antigen and TNF-α ( Fig. 2d,e ) was a clear difference in binding above background observed (44% binding, ~75% of that observed for positive control, Fig. 2d,e ; dark blue, pink). Variations with only one of the two inputs, antigen or TNF-α, ( Fig. 2e ) showed only background levels (<10%) of cellular detection by the AND-Ab. Notably, this conditional cellular detection by the AND-Ab was also visible by fluorescence microscopy ( Supplementary Figs 25,26 ), revealing cell-surface antigen sites and, thereby, also highlighting the potent utility of the AND-Ab system in direct imaging of cellular sites that generate two inputs within complex settings. Testing of the AND-Ab in Tissue This apparent ability of the AND-Ab to reveal such complex ‘two input’ cellular morphologies was next tested in mammalian tissue. First, cells expressing all various combinations of inputs were transplanted into mice through cranial injection into the left striatum as a putative model of diseases of the brain that can generate multiple biomarkers (8-week-old C57BL/6 mice). All cells were tested for positive generation of corresponding inputs before transplantation ( Supplementary Fig. 27 ). After 24 h, the ability to detect these cells in tissue was tested. Clear cellular detection, shown through fluorescence ( Supplementary Figs 28,29 ) was observed only for ‘dual input’ cells and at detection levels and with morphology essentially identical to those for positive controls ( Supplementary Fig. 28 ). In the absence of one or both inputs, the AND-Ab showed no cellular detection in tissue ( Supplementary Figs 28,29 ). Next, we tested the AND-Ab system’s response to a representative in vivo input that might indirectly trigger activity ( Fig. 3 and Supplementary Figs 30–32 ). Lipopolysaccharide (LPS) from Escherichia coli is a potent signal of pathogenic infection. LPS as a circulating in vivo input induced clear cellular detection ( Fig. 3 , bottom right) by the AND-Ab. Thus, through the use of a pathogen-associated input, here LPS, we were able to induce phosphatase expression using in vivo cytokine relay via endogenously-induced TNF-alpha that, in turn, led to ungating. Importantly, the AND-Ab showed no signs of either degradation or nonspecific dephosphorylation when incubated in plasma even for 24 h ( Supplementary Figs 33–35 ). Global assessment of phosphatase activities derived from homogenate of relevant organs of interest ( Supplementary Figs 36,37 ) also revealed the capacity for levels of activity sufficient for the application of the gated AND-Ab system in the kidney, brain, heart and lung. 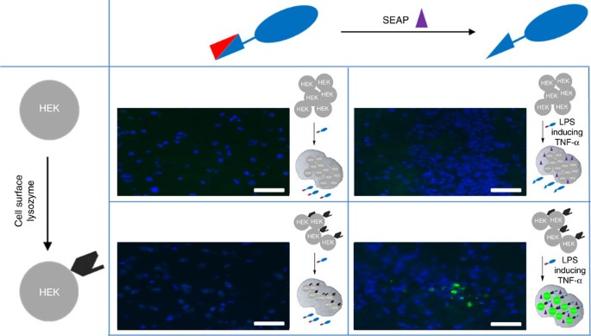Figure 3: Mammalian input activation of the AND-gated antibody. The gated antibody allowed ‘dual-input’-only imaging of mammalian brain tissue. After stimulation by the representative circulating pathogenic marker LPS, mice brains were generated containing cells expressing varying combinations of input states (no input, antigen-input only, phosphatase (SEAP, shown by a purple triangle in cartoons) input only and dual input). After overnight incubation, mice were killed and the brains sliced into 10 μm thick sections. Only dual input gave rise to output (fluorescent cells are observed, bottom right) from the gated AND-Ab. In this way, a circulating pathogenicin vivosignal indirectly created a key input for the activation of the gated antibody relayed via endogenous cytokine. Nuclei staining by DAPI (blue). Scale bar, 50 μm. DAPI, 4′,6-diamidino-2-phenylindole. Figure 3: Mammalian input activation of the AND-gated antibody. The gated antibody allowed ‘dual-input’-only imaging of mammalian brain tissue. After stimulation by the representative circulating pathogenic marker LPS, mice brains were generated containing cells expressing varying combinations of input states (no input, antigen-input only, phosphatase (SEAP, shown by a purple triangle in cartoons) input only and dual input). After overnight incubation, mice were killed and the brains sliced into 10 μm thick sections. Only dual input gave rise to output (fluorescent cells are observed, bottom right) from the gated AND-Ab. In this way, a circulating pathogenic in vivo signal indirectly created a key input for the activation of the gated antibody relayed via endogenous cytokine. Nuclei staining by DAPI (blue). Scale bar, 50 μm. DAPI, 4′,6-diamidino-2-phenylindole. Full size image Together, using model biomarker inputs, these data support the principle of an ‘AND antibody’ gated system that is applicable not only in vitro but also in mammalian cell systems and even in more complex mammalian tissue environments. The type of inherently gated protein system we create here would allow good transferability and ‘scalability’, a difficulty that surrounds some protein components [3] . Our use of antibody CDRs as control elements possesses the strong advantage of somatic mutation for their generation (a strong aid to rapid alteration and scalability) should new ‘gates’ be required. Notably in this study we utilized single-chain V H H camelid antibody constructs; these show particular strengths in ease of production, portability as genetic constructs and wide-ranging biotechnological application [23] . In particular, they display properties that might allow their particularly advantageous application, such as in intracellular applications under the control of cytosolic inputs in addition to the cell-surface inputs that we have shown here [24] , [25] . Nonetheless, the approach we describe here is a general one that is potentially applicable to conventional antibodies and ‘biologics’ in general. The AND-Ab system could therefore be considered for a wide range of roles in future medical applications: for example, to be a variant of some form of protected, ‘caged’ or pro-Ab, which is released upon triggering by the correct enzymatic activity. This may also be viewed as an artificial recapitulation of a dynamic posttranslational modification (here phosphorylation) but here in the service of a designed (rather than an evolutionary) goal. To the best of our knowledge, this is the first example of the use of chemical modification to temporarily inhibit/gate an antibody’s binding ability and then to restore it using an endogenous enzyme. Such systems, therefore, have strong potential for application in therapeutic systems where they could serve as ‘inhibited or pro-antibodies’ to target relevant cell-surface antigens [26] , [27] , [28] . The use of such gated antibodies could not only be used to block binding sites in antibodies but such a gated blocking technique could, in principle, be extended to any site where the presence of a functional group might have a modulating effect upon function (for example, through steric blockade or charge–charge interactions). Such sites could include enzyme-active sites that might be (allosterically) blocked, for instance, through such gating technology to prevent substrate utilization or these could also be sites in proteins that control essential conformation changes. It should also be noted that the methodology is not necessarily dependent on the phosphate-induced gating that we have proposed here but other groups (for example, glycosyl units) can also be introduced using the same technology and might then be utilized in systems that use other enzymes as the second gate input. In principle, therefore, such chemical modification is facile and could be applied to a number of other biochemically relevant but chemically installable groups such as sugars or peptides that might be cleaved by suitable glycosidases [29] , [30] and peptidases [28] , respectively. This creation of an artificial, but more stringent, antibody system may have application in minimizing side effects in a therapeutic context not only for therapeutic antibodies that act directly, but also for genetic Ab-protein fusions (bearing protein drugs or drug-releasing enzymes [31] ) and Ab-cytotoxin conjugates, where toxic side effects through insufficient targeting can present a strong current therapeutic hurdle [32] . As such, targeted systems can be envisaged for tumour treatment where matrix-degrading enzyme and tumour-associated marker (some of which are also found to some extent on normal tissue) could combine powerfully to overcome the limitations of just one of these markers alone. Timed-release Abs could be envisaged based on gated Abs that could avoid tachyphylaxis. Moreover, gated Abs could allow the ‘switching off’ of Ab treatment to avoid certain rare but known emergent side effects, such as progressive multifocal leukoencephalopathy. To date, no general strategy has been developed for the creation of discrete Boolean-gated proteins (for example, binding proteins such as Abs). Even when ‘proteins devices’ have been considered previously they have typically been used as codified functional inputs to gene networks rather than outputs in their own right [3] . One alternative elegant approach has used combinations of protein domain modules to build switchable proteins [33] . Although such multienzyme or multimodule systems may possess properties that allow them to mimic Boolean behaviours [34] , the design of an antibody-based state machine described here, in which input and output sites are colocalized in the CDR, valuably allows direct synchronization [35] of recognition function in a single molecule as the ‘computational element’ (see Supplementary Fig. 38 for the corresponding Boolean ‘truth table’ variants of Figs 1 , 2 , 3 ). The next stage for a generalized application of Boolean protein logic would be combination with other ‘gates’. Every Boolean calculation can be expressed using just two gates (AND and NOT or OR and NOT). Given that ‘cross-reactive’ or bi-specific [36] Abs can be considered to already operate with a Boolean OR logic, one can readily envisage more complex logic-gated-Ab processes. Following this first proof-of-principle study, the broader possible roles of these ‘logic-gated’ Abs (ANDibodies, Booleabodies) and their use for a new mode of ‘Boolean probing’ of multiple therapeutically relevant biomarkers and ‘Boolean-targeted’ delivery are ongoing in the group. Ultimately, the future therapeutic potential of the gated antibody strategy will rely on its behaviour within a given organism. Here, we show not only promising stability towards serum to allow AND-Ab dissemination but also that in the presence of a suitable marker enzyme, the antibody gets activated to bind displayed cell-surface antigen. In this way binding function is activated by two inputs; next steps towards therapeutic application should investigate therapeutic tasks beyond simply binding (for example, toxin delivery, cellular activation or pathogen neutralization). cAbLys3-pCys104 cAbLys3-Dha104 was synthesized using bisalkylative elimination of the corresponding cysteine mutant protein cAbLys3-Cys104 ( Supplementary Fig. 2 ) [8] . cAbLys3-Dha104 (980 μl, c=0.5 mg ml −1 in phosphate-buffered saline (PBS) pH 8) was concentrated down to 500 μl (Vivaspin, 5 K MWCO, Sartorius Stedim) and then split into five aliquots of 100 μl each. A solution of Na 3 SPO 3 (59 mg, 328 μmol) was made in 18.6 μl MQ H 2 O and 20 μl 5 M HCl. A total of 4 × 2.5 μl of the Na 3 SPO 3 solution (84.9 μmol, ~2,700 equivalent) was added to each aliquot over 30 min while shaking (600 r.p.m.) at 37 °C. The reactions were continued for 7 h in total, after which analysis by LC-MS revealed full conversion to cAbLys3-pCys104 (calculated (calc.) mass 15,874; observed (obs.) mass 15,875, Supplementary Fig. 3 ). The reaction solution was buffer exchanged and desalted using a PD10 minitrap. Cleavage of phosphate in cAbLys3-pCys104 A solution of human PLAP (1 mg, 1.3 U) in 50 μl 50 mM Tris-HCl pH 7.4 was prepared. A volume 17 μl of the enzyme solution (0.44 U) was added to cAbLys3-pCys104 (150 μl, 4.6 nmol, c=0.45 mg ml −1 in 50 mM Tris-HCl pH 7.4), and the reaction shaken at 37 °C (600 r.p.m.). After 2 h, LC-MS analysis revealed full conversion to cAbLys3-Cys104 (calc. mass 15,797; obs. mass 15,800, Supplementary Fig. 8 ). Ellman’s titration of cAbLys3-Cys104 A stock solution of Ellman’s reagent was prepared by dissolving 0.6 mg in 108 μl 10 mM PBS, pH 8.0. A 75 μl aliquot cAbLys3-Cys104 (c=0.5 mg ml −1 in 10 mM PBS, pH 8.0) was diluted with 75 μl 10 mM PBS, pH 8.0. A 10 μl aliquot of the Ellman’s reagent stock solution was added to the diluted protein. The solution was shaken at room temperature for 15 min. After this time, the reaction was analysed directly by LC-MS, and revealed full conversion to the Ellman’s adduct, confirming consumption of the thiol (calc. mass 15,994; obs. mass 15,992, Supplementary Fig. 13 ). Enzyme-linked immunosorbent assay Each well of a 96-well plate (Greiner Bio-One half-area high-binding plates) was coated with 1 μg of hen egg white lysozyme (Sigma), and incubated at 4 °C overnight. All subsequent steps were performed at room temperature. The plate was washed four times with PBS (pH 7.4) containing 0.05% TWEEN20 (Sigma), blocked for 90 min with 3% bovine serum albumin in PBS and then washed once with PBS (pH 7.4) containing 0.05% Tween20. Antibody (0.48 mg ml −1 in 1% BSA, 0.02% Tween20 in PBS) dilutions were made across the plate for final concentrations of 240 μg ml −1 to 234 ng ml −1 . The plate was incubated with gentle rocking for 2 h. Unbound antibody was removed by washing four times with PBS (pH 7.4) containing 0.05% Tween20. The secondary antibody (Anti-polyHistidine-alkaline phosphatase conjugate, Sigma) was prepared at a 1:1,000 dilution in PBS (pH 7.4) and 50 μl was added to each well. The plate was incubated with gentle rocking for 1 h. Each well was then washed with 50 μl of diethanolamine buffer (phosphatase substrate kit, Thermo Scientific). PNPP phosphatase substrate (phosphatase substrate kit, Thermo Scientific) was prepared by dissolving one tablet in 6 ml of diethanolamine buffer. A volume 50 μl of the PNPP substrate solution was added to each well and incubated for 15 min. After this time, absorbance was measured at 405 nm. Absorbance was plotted against concentration. Sigmoidal regression analysis and normalization was carried out using GraphPad Prism 5.01 ( Supplementary Fig. 14 ). Cell Culture Lysozyme (pIMMs2011LysD52S) under the CMV (cytomegalovirus) promoter was obtained from H. Finney (UCB). CMV-SEAP in pBluescript was obtained from Addgene (plasmid 24595). Human embryonic kidney (HEK293T) cells were cultured in Dulbecco’s modified Eagle’s Medium (DMEM, Life Technologies) supplemented with 10% (v/v) FBS (Sigma), 50 U ml −1 penicillin, 50 μg ml −1 streptomycin (Sigma) and 100 μg ml −1 Normocin (Invivogen) in a T25 flask (Greiner Bio-One). HEK-Blue Null1 cells (HEK-Blue Null1 (NF-kB- seap +), Invivogen) were cultured in DMEM supplemented with 10% (v/v) FBS, 50 U ml −1 penicillin, 50 μg ml −1 streptomycin, 100 μg ml −1 Normocin and 100 μg ml −1 Zeocin (Invivogen) in a T25 flask. All cells were maintained at 37 °C under 5% CO 2 with passaging every 3–4 days. Xfect transfection reagent was purchased from Clontech, PentaHis Alexa Fluor 488 from Qiagen, recombinant human TNF-α from Invivogen and recombinant mouse TNF-α from eBioscience. Xfect-mediated transfection of HEK293T cells with lysozyme and SEAP was carried out according to the manufacturers’ protocol. Accordingly, one day before transfection, cells were plated in 500 μl complete growth medium (in each well of a 12-well plate) to reach 50–70% confluency. After 24 h, plasmid (2.5 μg lysozyme or SEAP, in the case of co-transfections, 1.2 μg of each plasmid was used) was diluted with Xfect reaction buffer to a final volume of 50 μl and vortexed. Xfect Polymer was added to the diluted plasmid DNA (0.3 μl for every 1 μg plasmid) and vortexed. The polymer-plasmid solutions were incubated at room temperature for 10 min to allow nanoparticle complexes to form. A volume 50 μl of the nanoparticle complex solution was added dropwise to the cell culture medium (per well). Plates were rocked gently back and forth, and then incubated at 37 °C for 4 h. After this time, cell culture medium was replaced with 1 μl of fresh complete growth medium, and returned to 37 °C for approximately a further 40 h. For the induction of SEAP expression in HEK-Blue Null1- seap + cells, TNF-α was added to relevant wells at 100 ng ml −1 at approximately 24 h into expression. Antibody (WT-cAbLys3 or cAbLys3-pCys104) was added to relevant wells at 1 μM at approximately 28 h into expression. For SEAP detection, 18 μl test medium (containing 10% (v/v) heat-inactivated FBS) was added to wells of a 96-well plate, with 2 μl cell supernatant. 180 μl QUANTI-Blue (chromophoric phosphatase substrate) was added, and the plate incubated at 37 °C for 1–3 h, after which SEAP activity could be observed by the naked eye (pink–purple), and quantitatively determined using a spectrophotometer at 620 nm. After expression (~44 h), cells were washed three times with 500 μl of washing buffer (PBS+2% FBS) and incubated at room temperature with PentaHis Alexa Fluor 488 (0.5 μg ml −1 ) for 30 min. Cells were washed three more times with washing buffer, and then analysed by flow cytometry and microscopy. Ex vivo experiments HEK-Blue Null1 cells were transfected in a 12-well plate either with lysozyme (using pIMMs2011LysD52S ( lys ) or cultured in the absence of any transfection reagent. Forty-eight hours after transfection, media was removed. A sample was taken for confirmation of SEAP expression inducible by mouse TNF-α ( Supplementary Fig. 30a ). Cells were washed three times with DMEM (no additives) and lifted with 500 μl DMEM and counted. An aliquot of 10 4 cells was taken to test for lysozyme expression ( Supplementary Fig. 30b ), and a sample containing 10 6 cells was spun down (5 mins, 1.2 k.r.p.m.). Supernatant was removed and the cell pellet resuspended in 2 μl DMEM. In vivo Eight-week-old male C57BL/6 mice (Harlan, UK) were allowed to acclimatize for 7 days before injection. All surgical procedures were performed under an operating microscope (Wild M650, Leica, Milton Keynes, UK) with UK Home Office and local ethical approval. Animals were anaesthetised with isoflurane (Rhodia Organique Fine Ltd, Bristol, UK) for induction and maintenance at 2.5–3% in oxygen. Stereotaxic surgery was performed as described previously [37] . A total of 0.5 ml (10 μg μl −1 ) LPS ( E. coli 026:B6, Sigma-Aldrich) or saline vehicle was injected via finely-drawn glass microcapillaries as previously described [38] . Then, anaesthetised mice were held in a stereotaxic frame, a burr hole was drilled in the skull and a 2 μl volume of the cell suspension was unilaterally microinjected into the left striatum through a glass microcapillary needle over a period of 5 min. The stereotaxic co-ordinates were: bregma +0.5 mm, lateral 1.8 mm, and the cells were injected from a rising depth of 2.5–1.5 mm. During the surgical procedures, body temperature was maintained on a heated blanket throughout the period of anaesthesia, and the animals were allowed to recover in a heated chamber. Mice were killed after 24 h by deep anaesthetic with sodium pentobarbitone and transcardial perfusion with cold saline (4 °C). Brains were frontally cut into 10 μm thick cryostat sections through the injection site onto RNAse free Super Frost Plus slides (Thermo Scientific, Germany). Tissue slices on slides were removed from −20 °C and 50 μl blocking buffer (50 mM Tris–HCl pH 7.4, 2% mouse serum, 0.01% TWEEN20) was added to immerse each tissue slice in a well constructed with a PAP pen for immunostaining. Blocking was allowed to occur for 10 min at room temperature after which it was replaced with antibody solution (1 μM in blocking buffer). Slide-mounted tissue was incubated at 37 °C 5% CO 2 in a humidity chamber for 2 h. As a positive control, WT-cAbLys3 was added to a single tissue section injected with HEK-Blue Null1- lys + cells ( Supplementary Fig. 31 ). Slides were washed to remove excess antibody by dipping in a beaker of 50 mM Tris–HCl pH 7.4 10 times and then each tissue slice fixed with 50 μl 4% formaldehyde for 5 min at room temperature, and then washed three times. Blocking was repeated for 10 min at room temperature. PentaHis Alexa Fluor 488 in blocking buffer (0.5 μg ml −1 ) was added to each slice in the humidity chamber and staining was allowed to occur for 1 h at room temperature. Again, slides were dipped 10 times into 50 mM Tris-HCl pH 7.4 to remove excess antibody. Excess liquid was removed from the slides with a medical wipe, each slice was covered with a coverslip containing one drop of mounting medium (with 4′,6-diamidino-2-phenylindole) and allowed to harden overnight at 4 °C. Immunostained sections were tested for fluorescence by microscopy. How to cite this article : Gunnoo, S. B. et al. Creation of a gated antibody as a conditionally functional synthetic protein. Nat. Commun. 5:4388 doi: 10.1038/ncomms5388 (2014).